Sn-Beta zeolites with borate salts catalyse the epimerization of carbohydrates via an intramolecular carbon shift Carbohydrate epimerization is an essential technology for the widespread production of rare sugars. In contrast to other enzymes, most epimerases are only active on sugars substituted with phosphate or nucleotide groups, thus drastically restricting their use. Here we show that Sn-Beta zeolite in the presence of sodium tetraborate catalyses the selective epimerization of aldoses in aqueous media. Specifically, a 5 wt% aldose (for example, glucose, xylose or arabinose) solution with a 4:1 aldose:sodium tetraborate molar ratio reacted with catalytic amounts of Sn-Beta yields near-equilibrium epimerization product distributions. The reaction proceeds by way of a 1,2 carbon shift wherein the bond between C-2 and C-3 is cleaved and a new bond between C-1 and C-3 is formed, with C-1 moving to the C-2 position with an inverted configuration. This work provides a general method of performing carbohydrate epimerizations that surmounts the main disadvantages of current enzymatic and inorganic processes. Carbohydrate chemistry is a critical enabling technology for numerous processes in the health, food, chemical and alternative fuel industries. Of all possible pentoses and hexoses, only seven (that is, D -glucose, D -galactose, D -mannose, D -fructose, D -xylose, D -ribose and L -arabinose) are found in nature in sufficient amounts to allow their commercial production, while all others are denominated as 'rare' [1] . Despite their low natural abundance, rare sugars have enormous potential in several important applications, including their use as components for antiviral drugs [2] , low-calorie sweeteners with low glycemic indexes [3] , anti-inflammatory agents with immunosuppressive properties [4] and chiral building blocks in natural products synthesis [5] . Biochemical processes are primarily employed to transform abundant sugars into rare ones using three main classes of enzymes, namely keto-aldol isomerases, epimerases and oxidoreductases (see Fig. 1 ). Isomerases and oxidoreductases are widely used because they are active on a wide range of simple substrates; however, such general activity is not always an advantage because it can result in the formation of side products (for example, xylose isomerase converts glucose into fructose and simultaneously converts fructose into mannose). These processes have generated some commercially available rare sugars (for example, D -sorbose and D -tagatose), but in most cases the complex nature of the bio-chemical process coupled with the thermodynamic limitations associated with sugar conversions performed at a strict upper bound temperature makes the synthesis and purification of rare sugars costly. In this respect, epimerases are potentially the most useful biocatalysts for the widespread production of rare sugars. They offer high specificity for products and are capable of selectively modifying sugars at multiple carbon positions (unlike isomerases, which are restricted to modifications of C-1 and C-2 positions) [6] . For example, a 2-epimerase could replace the double keto-aldol isomerization required to convert D -xylose into D -lyxose. Unfortunately, most epimerases (with the notable exception of D -tagatose 3-epimerase) are only active on sugars that are substituted with phosphate or nucleotide groups, thus drastically restricting their use. 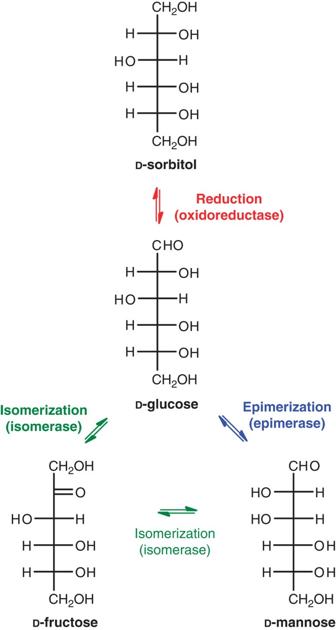Figure 1: Representative glucose conversion pathways using biological catalysts. Enzymes comprise isomerases, oxidoreductases and epimerases. Figure 1: Representative glucose conversion pathways using biological catalysts. Enzymes comprise isomerases, oxidoreductases and epimerases. Full size image Inorganic catalysts can provide alternative chemical pathways to those offered by biological systems. In contrast to enzymes, inorganic catalysts function over a larger range of reactant purities, temperatures, pressures and pH. For equilibrium-limited endothermic reactions, the ability to function at higher temperatures allows for operation in a regime where the equilibrium is more favorable. In addition, solid catalysts, such as zeolites, are easily separated from gas- or liquid-phase reactions and can be readily regenerated by calcination upon deactivation. The performance of the current generation of inorganic catalysts rarely matches that of their enzymatic counterparts; however, newly developed inorganic catalysts that have activities and selectivities comparable to those of enzymes will provide more efficient isomerization, epimerization and oxidation/reduction routes. This will increase the availability of rare sugars for the discovery and implementation of new applications. Tin-containing silicates have recently emerged as a new class of inorganic solids with Lewis acid character capable of activating carbonyl functional groups in the presence of water [7] . The pioneering work by Corma et al . [8] , [9] , [10] , [11] showed that Sn-Beta (that is, a zeolite with the Beta topology containing a small weight percent of tin present as isolated sites tetrahedrally coordinated in the zeolite framework) is highly active in Meerwin–Ponndorf–Verley (MPV) reduction and Baeyer–Villiger oxidation reactions. In contrast to most Lewis acids that require strictly anhydrous conditions, Sn-Beta remained active in the presence of small amounts of water. For the MPV reaction between alcohols and ketones, Corma et al . [10] showed that Sn incorporated in the framework of zeolite Beta has adequate Lewis acidity to polarize the carbonyl group in the ketone while providing open coordination sites for both the ketone and the alcohol. Davis et al . [12] , [13] , [14] have recently demonstrated that Sn-Beta is active in the isomerization of sugars in bulk water and showed that it operates via chemical pathways analogous to those observed in isomerases. Sn-Beta and other tin-containing silicates have also been used for the isomerization of trioses in organic media to produce lactate derivatives [15] , [16] , [17] , [18] , [19] . Here we show that zeolites containing isolated Lewis acid sites used in conjunction with borate salts catalyse the epimerization of carbohydrates in a cooperative manner. This catalytic system is robust, featuring high activity and selectivity for the conversion of various aldoses over a broad range of reaction conditions. For example, a system comprising Sn-Beta and sodium tetraborate (SB) (molecular formula Na 2 [B 4 O 5 (OH) 4 ]·8H 2 O) epimerizes aldoses to an equilibrium mixture containing the reactant (for example, glucose, xylose or arabinose) and the epimer (for example, mannose, lyxose and ribose, respectively), without producing significant quantities of the ketose isomer (for example, fructose, xylulose and ribulose, respectively). We demonstrate that borates have a critical role in stabilizing the intermediate required for Sn-Beta to catalyse the epimerization by way of a 1,2 intramolecular carbon shift, whereby C-1 and C-2 undergo a transposition such that the former C-1 takes the place of C-2 with an inverted configuration. This drastically differs from the typical use of borates to shift the thermodynamic equilibrium through LeChatlier's principle by preferentially complexing with the ketose products [20] . The present work demonstrates a simple, general route for the epimerization of carbohydrates using solid Lewis acid catalysts. This catalytic system features activities and selectivities resembling those of epimerases, while also overcoming many of the drawbacks associated with biocatalytic processes. Reactivity data Glucose reactivity data obtained with the combined use of Sn-Beta and SB show that both constituents are needed to achieve the epimerization of glucose to mannose. Specifically, when a 4:1 glucose:SB solution is used in the presence of Sn-Beta at a temperature of 358 K for 60 min, a product distribution of 84:1:15 glucose:fructose:mannose (99% of the total carbon) is generated (see Table 1 , entry 4). On the contrary, when the reaction is performed under identical conditions but in the absence of borate, an 83:16:1 glucose:fructose:mannose (95% of the total carbon) distribution is obtained that is consistent with the product distribution previously reported for glucose isomerization using Sn-Beta (see Table 1 , entry 5) [12] . Additional control experiments show that under the temperature and reaction times investigated, glucose is unreactive in SB solutions or in SB solutions containing pure silica Beta zeolite (see Table 1 , entries 1 and 2). We note that similar results are obtained for other aldoses (see Table 1 , entries 7–14). Thus, starting from D -xylose, a 75:3:22 xylose:xylulose:lyxose (93% of total carbon) product distribution was obtained with SB, as compared with a distribution of 79:13:8 (96% of total carbon) in the absence of borate, and starting from D -arabinose with SB, a 68:1:31 arabinose:ribulose:ribose (97% of total carbon) product distribution was obtained as compared with 84:11:5 (83% of total carbon) in the absence of borate. Time studies for glucose, xylose and arabinose are shown in Supplementary Tables S1–S3 . Table 1 Results for the isomerization/epimerization of sugars. Full size table Reaction mechanism To gain insight into the epimerization reaction mechanism, isotopically labeled glucose was reacted with the Sn-Beta/SB system and investigated using 13 C nuclear magnetic resonance (NMR). Before reaction, a 5 wt% D -(1- 13 C)glucose solution containing SB in a 4:1 glucose:SB molar ratio generates resonances at δ =97.0 and 93.2 ppm, as well as a multiplet at δ =103.4–104.5 ppm (see Fig. 2a ). The first two resonances correspond to the C-1 carbon of the β-pyranose and α-pyranose configurations of glucose, respectively, and the multiplet is consistent with the chemical shifts induced on C-1 by complex formation between the borate anion and the hydroxyl group at C-1 (ref. 21 ). Previous reports have shown that SB readily interacts with molecules containing vicinal diols, forming stable monomeric and dimeric boroxy species [22] . 11 B and 13 C NMR spectra for sugars dissolved in the presence of SB confirm the presence of monomeric and dimeric sugar–boron complexes (see Supplementary Tables S4 and S5 and Supplementary Figs S1–S9 ). After reaction, a new set of resonances appear at δ =71.8 and 72.3 ppm (see Fig. 2b ). Surprisingly, these resonances correspond to the two chemical shifts of D -(2- 13 C)mannose that are separated by ~0.5 ppm due to vicinal C–C coupling interactions with the α and β forms of the anomeric carbon [23] . Fractionation of the reaction mixture using high-performance liquid chromatography (HPLC) followed by 13 C and 1 H NMR analyses of the product fraction confirm the identity of the products (see Supplementary Figs S10 and S11 ). These results indicate that a rearrangement of the carbon backbone occurred, with C-1 and C-2 exchanging positions by way of an intramolecular carbon shift where the bond between C-2 and C-3 is cleaved and a new bond between C-1 and C-3 is formed. To obtain the epimer, the former C-1 atom (now at the C-2 position) must have an inverted configuration and the process has to be accompanied by hydride transfer steps at O-1 and O-2. An isotopic effect was not observed when the reaction was performed in deuterium oxide (D 2 O), suggesting that H-D exchange processes are not involved in the kinetically relevant steps. 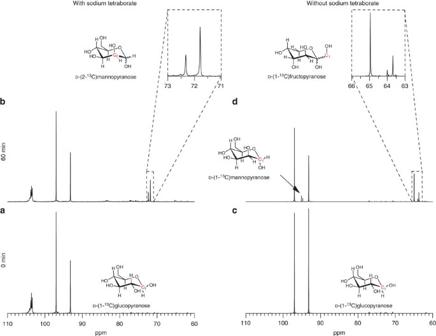Figure 2:13C NMR spectra of reactants and products for epimerization and isomerization reactions. (a)D-(1-13C)glucose with SB in a 4:1 glucose:SB ratio; (b) product mixture after reactingD-(1-13C)glucose with SB in a 4:1 glucose:SB ratio and Sn-Beta; (c)D-(1-13C)glucose; and (d) product mixture after reactingD-(1-13C)glucose with Sn-Beta. Figure 2: 13 C NMR spectra of reactants and products for epimerization and isomerization reactions . ( a ) D -(1- 13 C)glucose with SB in a 4:1 glucose:SB ratio; ( b ) product mixture after reacting D -(1- 13 C)glucose with SB in a 4:1 glucose:SB ratio and Sn-Beta; ( c ) D -(1- 13 C)glucose; and ( d ) product mixture after reacting D -(1- 13 C)glucose with Sn-Beta. Full size image A similar 13 C NMR study performed under identical reaction conditions but in the absence of borate generates drastically different results. Before reaction, only the two resonances at δ =97.0 and 93.2 ppm are observed for the 5 wt% D -(1- 13 C)glucose solution (see Fig. 2c ). After reaction, two new sets of resonances appear: the first set at δ =63.7 and 65.0 ppm corresponding to the α-furanose and β-pyranose conformations of D -(1- 13 C)fructose and the second set at δ =94.6 and 95.1 ppm corresponding to the β-pyranose and α-pyranose configurations of D -(1- 13 C)mannose (see Fig. 2d ). Evidently, when the reaction is catalysed by Sn-Beta without borates, no carbon backbone rearrangement occurs and the reaction proceeds by way of an intramolecular hydride shift as reported in previous studies [13] . Sugar–borate complex To determine the role borate–sugar complex formation has on product distribution, a series of reactions varying the SB content were performed. As shown in Table 2 , decreasing SB content results in a shift in the product distribution from mannose to fructose, while addition of stoichiometric or higher amounts of borate yields virtually no fructose. This indicates that epimerization and isomerization processes occur competitively. Note that the epimerization is still dominant with sub-stoichiometric amounts of borate, suggesting that the sugar–borate complex is not permanent and could form preferentially within the pores of the zeolite. Additional experiments showed that pretreating the catalyst with borate before adding the sugar or premixing the sugar with borate before adding Sn-Beta did not affect these results. Table 2 Results for the isomerization/epimerization of sugars. Full size table Solid-state magic-angle spinning (MAS) 13 C and 11 B NMR spectra reveal that the sugar–borate complex exists inside the pores of the zeolite (see Fig. 3 ). Specifically, Sn-Beta was mixed with a D -(1- 13 C)glucose solution containing SB (with molar ratios of 2:0.5:1 and 100:25:1 D -(1- 13 C)glucose:SB:Sn for 13 C and 11 B, respectively) for 30 min at room temperature and then separated by vacuum filtration. The 13 C MAS NMR spectrum of the filtered Sn-Beta contains a set of resonances at δ iso ≈103 ppm that is consistent with the formation of glucose–borate complexes. Similar outcomes are observed in spectra obtained post reaction in the presence of SB. When the D -(1- 13 C)glucose solution does not contain SB or when SB is adsorbed in the absence of glucose, the resonances at δ iso =103 ppm are not observed. In addition, 11 B MAS NMR of the D -(1- 13 C)glucose sample adsorbed on Sn-Beta in the presence of SB shows the characteristic four-coordinate 11 B resonances associated with sugar–borate complex formation. Specifically, we observe one three-coordinate 11 B resonance centered at δ =17 ppm that is correlated with a disordered borate moiety likely due to the presence of free SB and four four-coordinate 11 B resonances centered at δ iso =11, 5.5, −0.5 and −4 ppm. The broad lineshapes observed for all the three-coordinate 11 B environments are due to a significant quadrupolar coupling constant of ~2.5 MHz and a low-asymmetry parameter ( η <0.2). In crystalline systems such as SB, a clean second-order quadrupolar pattern is observed ( C Q =2.53 MHz, η =0.09 and δ iso =19.8 ppm); however, in a disordered solid this will cause a broadening of the resonance into a Gaussian-like lineshape as seen for SB adsorbed on Sn-Beta and D -(1- 13 C)glucose with SB adsorbed on Sn-Beta (see Fig. 3e–g ) [24] . This phenomenon is not the case for the higher-symmetry four-coordinate 11 B resonances. The reduction in second-order quadrupolar broadening occurs due to the local symmetry being pseudo-tetrahedral (quadrupolar couplings on the order of a few 100 kHz), resulting in a near-isotropic lineshape. Of the four four-coordinate 11 B resonances, only the one at δ iso =−0.5 can correspond to B–O–B (that is, re-arrangement within SB) and B–O–Si (that is, Sn-Beta and SB interactions) environments [25] , [26] . These assignments are further confirmed by the 11 B MAS NMR spectrum of SB adsorbed on Sn-Beta (see Fig. 3f ), which exhibits a broad three-coordinate 11 B resonance and a narrower four-coordinate 11 B resonance centered at δ iso =0.5 ppm and a shoulder at δ iso =−0.5 ppm The concentration of possible B–O–Sn environments is too low to be detected with the current analytical method; therefore, the remaining four-coordinate 11 B resonances must correspond to sugar–borate complexes. Note that these resonances match those observed for glucose–borate complexes present in solution (see Supplementary Fig. S1 ). 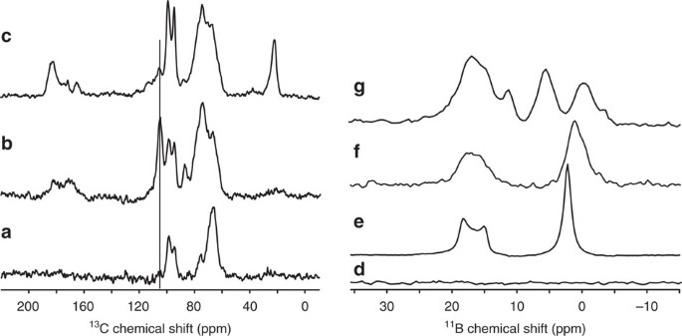Figure 3:13C and11B solid-state MAS NMR spectra for glucose adsorbed on Sn-Beta. (a)13C MAS NMR cross-polarization (CP) ofD-(1-13C)glucose adsorbed on Sn-Beta with a 2:1 glucose:Sn molar ratio; (b)13C MAS NMR (CP) ofD-(1-13C)glucose with SB in a 2:0.5:1 glucose:SB:Sn molar ratio; (c)13C MAS NMR (CP) ofD-(1-13C)glucose with SB after reaction at 358 K for 30 min with a 50:12.5:1 glucose:SB:Sn molar ratio; (d)11B MAS NMR of Sn-Beta; (e)11B MAS NMR of SB; (f)11B MAS NMR of SB adsorbed on Sn-Beta with a 12.5:1 SB:Sn molar ratio; and (g)11B MAS NMR ofD-(1-13C)glucose with SB adsorbed on Sn-Beta in a 2:0.5:1 glucose:SB:Sn molar ratio. Figure 3: 13 C and 11 B solid-state MAS NMR spectra for glucose adsorbed on Sn-Beta . ( a ) 13 C MAS NMR cross-polarization (CP) of D -(1- 13 C)glucose adsorbed on Sn-Beta with a 2:1 glucose:Sn molar ratio; ( b ) 13 C MAS NMR (CP) of D -(1- 13 C)glucose with SB in a 2:0.5:1 glucose:SB:Sn molar ratio; ( c ) 13 C MAS NMR (CP) of D -(1- 13 C)glucose with SB after reaction at 358 K for 30 min with a 50:12.5:1 glucose:SB:Sn molar ratio; ( d ) 11 B MAS NMR of Sn-Beta; ( e ) 11 B MAS NMR of SB; ( f ) 11 B MAS NMR of SB adsorbed on Sn-Beta with a 12.5:1 SB:Sn molar ratio; and ( g ) 11 B MAS NMR of D -(1- 13 C)glucose with SB adsorbed on Sn-Beta in a 2:0.5:1 glucose:SB:Sn molar ratio. Full size image X-ray photoelectron spectroscopy (XPS) data of Sn-Beta samples containing adsorbed species show both an increase in the amount of carbon on the surface and changes in the chemical nature of surface tin sites (see Supplementary Fig. S12 ). Specifically, calcined Sn-Beta showed doublets for Sn 3d 5/2 and 3d 3/2 electrons with binding energies of 487.2 and 495.6 eV, respectively, which is indicative of Sn 4+ species on the surface. Spectra for Sn-Beta containing adsorbed glucose and glucose/borate show a downward shift in the binding energy for the Sn 3d signal of ~0.3 and 0.9 eV, respectively. Also, these samples show an increase in the binding energy for the C 1s signal when compared with freshly calcined Sn-Beta. To gain further insight into the nature of the interaction between the sugar–borate complex, the zeolite pore and the active site, the epimerization of sugars with Sn-MCM-41 and Sn-MFI, which are stannosilicates with pore topologies different from Beta, was investigated. Interestingly, the epimerization-promoting effect of SB was only slightly detected for Sn-MCM-41 and not observed for Sn-MFI. For experiments performed with Sn-MCM-41 at 383 K with a 4:1 glucose:SB molar ratio, the product distributions in the presence and absence of SB are 76:11:13 (81% of total carbon) and 93:6:1 (99% of total carbon), respectively (see Table 2 , entries 5 and 8). Sn-MFI experiments with glucose did not show reactivity, but this is consistent with the fact that glucose is too large to enter the pores of MFI (see Table 2 , entries 6 and 9). Using xylose as the starting reagent, the product distributions in the presence and absence of SB are 84:12:4 and 79:15:6 xylose:xylulose:lyxose with sugar yields of 95% and 97%, respectively (see Table 2 , entries 11 and 12). In contrast, xylose reacted with Sn-Beta and SB is almost exclusively converted into lyxose (see Table 1 , entries 7 and 9). The results of the present study indicate that zeolites containing isolated Lewis acid sites and borate salts cooperatively catalyse the epimerization of carbohydrates. Base catalysts are typically used to produce epimers following Lobry de Bruyn-Alberda van Ekenstein pathways that produce mixtures of the ketose isomer and the aldose epimer via ene-diol transition states [27] . A rare exception to this mechanism was discovered by Bílik, who showed that treatment with catalytic amounts of molybdic acid under acidic conditions will epimerize aldoses via transition states that promote a 1,2 carbon shift [28] . Many catalytic systems based on molybdate chemistry have been investigated [29] , [30] . The accepted mechanism involves the complex formation of a binuclear molybdate species with four adjacent hydroxyl groups (OH-1 to OH-4) in the sugar [31] , [32] . The molybdate species creates a rigid framework that holds the atoms in the required conformation to promote the concerted C-3 bond migration from C-2 to C-1. Similar results have been reported for homogeneous Ni 2+ complexes with diamine co-catalysts in methanolic solutions [33] . In all cases, a rigid metal–sugar complex was required to achieve the carbon backbone rearrangement. In the present study, NMR investigations on isotopically labeled sugars show that the epimerization occurs via a 1,2 intramolecular carbon shift, which is similar to the mechanism proposed for the Bílik reaction catalysed by molybdate species. The borate–sugar complexes likely have a critical role in providing a rigid framework for the carbon shift to occur at the active site in the zeolite. This rigid complex facilitates bond bending to bring C-1 and C-3 close enough to promote bond migration. The data suggest that a synergistic effect between the pore walls of Beta, the isolated Lewis acid sites and the sugar–borate complex has to exist for the epimerization reaction to occur selectively. The 13 C and 11 B MAS NMR data show that the complex is likely present inside the pores of Sn-Beta and the XPS data indicate that adsorbed components change the electronic environment of the Sn surface sites. The inferior epimerization performance of other pore topologies suggests the presence of a strong confining effect in the 12-membered rings of Beta. We hypothesize that the large pores of Sn-MCM-41 allow all molecules, complexed and uncomplexed, to reach and react at the active site without restriction to generate a mixture of epimers and isomers. Conversely, the pores of Sn-MFI are too small for the sugar–borate complex to enter or form inside them, but are large enough to allow uncomplexed sugar to enter and undergo normal isomerization reactions at the tin site. In Sn-Beta, the borate may preferentially reside inside the pores, form the sugar–borate complex and preferentially absorb in the pores, or form a unique complex with both the sugar and the tin site. The present reaction and NMR data cannot conclusively exclude any of these options, thus requiring further studies. We note that the epimerization chemistry is not restricted to tin-containing zeolites. Experiments with Ti-Beta using glucose under standard reaction conditions showed that this catalyst had much lower activity than Sn-Beta, but generated a similar product distribution in the presence (87:0:13 glucose:fructose:mannose) and absence (92:6:2 glucose:fructose:mannose) of SB, with carbon balances exceeding 88% (see Table 2 , entries 7 and 10). The combination of Sn-Beta and SB generates a highly active catalytic system for epimerization reactions that, unlike most epimerases, can be used to process a variety of sugars to the thermodynamic equilibrium limit (see Table 1 for calculated equilibrium compositions) without the need of prior substrate functionalization. Currently, heterogeneous catalysts containing immobilized molybdate species in ion-exchange resins represent the state-of-the-art in sugar epimerization chemistry [34] . These inorganic catalysts have been optimized to minimize deactivation; however, slow and continuous leaching of the active phase is always observed and this effect is expected to increase in the presence of dissolved anions in the feed (for example, as those encountered in lignocellulosic biomass feedstock) [34] . The Sn-Beta/SB system is stable and active in the presence of high ionic strength solutions, thus offering an attractive alternative to process 'dirty' carbohydrate feeds containing dissolved anionic species that would foul catalysts based on ion-exchange resins. Importantly, the zeolite component can provide interesting reactivity pathways based on confining and shape selectivity effects induced by the micropores that are unattainable by ion-exchange resins. Future studies geared at designing catalytic sites that allow the formation of an immobilized rigid sugar–borate complex within the zeolite pores will be critical to reduce the number of separation unit operations by eliminating the use of complexing agents in solution. Finally, having observed C–C bond-breaking and bond-forming events associated with rigid sugar complexes activated with Sn-Beta, it is anticipated that this catalytic system may be applied to other classes of oxygenated molecules and more general reactions. We are intrigued by the potential links between the observed carbon backbone rearrangement and C–C bond-forming events in prebiotic chemistry. For instance, the formose reaction involves the bottom-up synthesis of pentoses and hexoses by a series of borate- or silicate-stabilized formaldehyde coupling sequences [35] , [36] , [37] , while the 'glyoxylate scenario' proposes glyoxylate and dihydroxyfumarate intermediates for forming carbohydrates in the presence of Lewis acidic salts [38] , [39] . Understanding such C–C coupling in carbohydrates is currently the subject of additional studies within our group. Synthesis of Sn-Beta Sn-Beta was synthesized according to Corma et al . [40] , as follows: 24.67 g of aqueous tetraethylammonium hydroxide (Sigma-Aldrich, 35% (w/w)) and 22.14 g of tetraethylorthosilicate (Sigma-Aldrich, 99% (w/w)) were added to a Teflon ® (Polytetrafluoroethylene, [PTFE]) dish, which was stirred at room temperature for 90 min. Then, 0.380 g of tin (IV) chloride pentahydrate (Sigma-Aldrich, 98% (w/w)) dissolved in 15 g of deionized water (DI H 2 O) was added dropwise. The solution was left uncovered on a stir plate for 10 h to reach 15 g of total water. Next, 2.407 g of aqueous hydrofluoric acid (Sigma-Aldrich 48% (w/w)) was added dropwise and the mixture was homogenized using a PTFE spatula, resulting in a thick gel. Then, 0.333 g of previously made Sn-Beta was seeded into the mixture, which was allowed to evaporate to a final molar composition of SiO 2 /0.01 SnCl 4 /0.55 TEAOH/0.54 HF/7.52 H 2 O. The thick paste was transferred to a PTFE-lined stainless steel autoclave and heated to 413 K for 40 days. The solids were recovered by filtration, washed with DI H 2 O, dried at 373 K and calcined at 853 K for 10 h with a 1-K min −1 ramp and 1 h stops at 423 and 623 K, leading to an overall inorganic oxide yield of 80–90%. Powder X-ray diffraction (PXRD) confirmed that the solid material has the Beta zeolite topology (see Supplementary Fig. S13 ). The ultraviolet–visible diffuse reflectance spectrum of the calcined sample shows the presence of a unique band at ~200 nm, which has been associated with Sn tetrahedrally coordinated into the zeolite framework (see Supplementary Fig. S14 ). A scanning electron microscopy (SEM) image is shown in Supplementary Figure S15 and SEM energy-dispersive X-ray spectroscopy (EDS) measurements show an atomic ratio Si:Sn of 110:1. This result is consistent with the Si:Sn of 111:1 obtained from elemental analysis (Galbraith Laboratories, Inc). Ti-Beta was synthesized in a similar way as described in the Supplementary Methods, with an XRD shown in Supplementary Figure S16 . Synthesis of other stannosilicates Sn-MFI was synthesized according to Mal et al . [41] , as follows: 0.098 g of tin (IV) chloride pentahydrate (Sigma-Aldrich, 98% (w/w)) was added to 5 g of DI H 2 O in a PTFE dish. Further, 8.350 g of tetraethylorthosilicate (Sigma-Aldrich, 99% (w/w)) was added and the solution was stirred for 30 min. Then, 8.966 g of aqueous tetra- n -propyl ammonium hydroxide (Alfa Aesar, 20%(w/w)) was added and the mixture was stirred uncovered for 1 h. Next, 20.083 g of DI H 2 O was added and the solution was allowed to mix for 30 min to a final synthesis gel molar composition of SiO 2 /0.01 SnO 2 /0.44 TPAOH/34.3 H 2 O. The solution was transferred to a PTFE-lined stainless steel autoclave and heated to 433 K for 48 h. After this time, the solids were repeatedly centrifuged and washed with DI H 2 O, dried at 373 K, and calcined at 853 K for 10 h with a 1 K min −1 ramp and 1 h stops at 423 and 623 K, leading to an overall 70–90% yield. PXRD confirmed that the solid material has the MFI zeolite topology (see Supplementary Fig. S17 ). The ultraviolet–visible diffuse reflectance spectrum indicates Sn is in the framework (see Supplementary Fig. S18 ). SEM EDS measurements for the Sn-MFI sample show an atomic ratio Si:Sn of 180:1. Please refer to the Supplementary Methods for a detailed description of the Sn-MCM-41 synthesis method. Catalytic reactions Catalysts were added at a 1:100 metal:sugar molar ratio to a 5 wt% sugar solution in a 5-ml thick-walled glass reactor containing a small magnetic stir bar (typically ~40 mg of catalyst in 2 ml of sugar solution). After taking a sample for t =0, the vial was sealed using a PTFE/silicone septa and metal crimp top, placed in a temperature-controlled oil bath and samples were taken at various times. After quenching the vial for 5 min in an ice bath, a small sample was removed using a syringe and filtered into a small vial. Next, 100 μl of the filtered sample and 20 μl of a 10 wt% mannitol solution were mixed in an HPLC vial. The samples were analysed on an Agilent 1260 HPLC system equipped with photodiode array ultraviolet and evaporative light-scattering detectors. The reaction products were separated using a Bio-Rad Aminex HPX-87C column heated to 353 K with DI H 2 O (pH=7) as the mobile phase at a flow rate of 0.6 ml min −1 . Xylulose and ribulose concentrations were determined using the ultraviolet detector at 210 nm. At this wavelength all other sugars had negligible ultraviolet signals. For all ultraviolet-inactive carbohydrates, the analysis was performed using the evaporative light scattering detector and Origin software (OriginLab Corp., ver. 9) for peak deconvolution when needed. The peak deconvolution function is based on Gaussian/Lorentzian fitting functions that provided an accuracy of ~8% when compared with standard mixtures. Sugar adsorption For the sugar adsorption studies, 100 mg of Sn-Beta was mixed with a 0.01-g ml −1 sugar solution (2:0.5:1 or 100:25:1 D -(1-13C)glucose:SB:Sn) for 30 min at room temperature and then quickly separated by vacuum filtration and dried under vacuum at room temperature. Post-reaction catalysts were produced in a similar way starting with a 0.05-g ml −1 sugar solution (50:1 D-(1-13C)glucose:Sn) and heating the mixture to 358 K for 30 min. Characterization PXRD patterns were collected using a Bruker D8 diffractometer with Cu Kα radiation. SEM EDS measurements were recorded on a JEOL 6700F at an electron high tension of 10 kV. Ultraviolet–Vis measurements were recorded using a Cary 3G spectrometer with a diffuse reflectance cell after calcination without subsequent drying. Nitrogen adsorption/desorption experiments were performed on a Quantachrome Autosorb iQ apparatus. Solution NMR was performed on a Bruker AVANCE 400 MHz spectrometer with a Magnex magnet and 5 mm double-resonance probe, which was tuned to 1 H, 11 B and 13 C before use. Samples were prepared at a sugar concentration of 0.05 g ml −1 using quartz NMR tubes. The spinning frequency was 20 Hz. For 1 H and 11 B 64 transients were taken, and for 13 C between 1024 and 2048 transients were taken. 1 H NMR spectra were referenced with respect to residual water. 13 C was referenced with respect to the C-1 carbon of D -glucose at 97.0 ppm as a secondary standard relative to 4,4-dimethyl-4-silapentane-1-sulphonic acid. All 11 B spectra were referenced using boric acid (H 3 BO 3 , 19.6) as a secondary standard relative to boron trifluoride etherate (BF 3 EtO 2 ). 13 C solid-state MAS NMR experiments were measured using an 11.7-T ( 1 H, 500.057 MHz) Magnex magnet and a home-built spectrometer (courtesy of Dr David Ruben, FBML-MIT). Experiments were performed using a 4-mm Varian-Chemagnetics MAS triple-resonance probe, doubly tuned to 13 C and 1 H. Powdered samples were packed into 4 mm outside diameter (o.d.) ZrO 2 rotors equipped with Vespel drive-caps and Kel-F top-caps. All 13 C spectra were acquired using two second recycle delays, a spinning frequency of ω r /2 π =9.00 kHz, and between 10 240 and 35 840 co-added transients. 13 C{ 1 H} cross-polarization [43] experiments were acquired using γB 1 of 50 kHz on 1 H and an optimized 13 C ramp with high-power 1 H decoupling (Two-pulse phase-modulated [TPPM] [44] , γB 1 of 83 kHz). All 13 C spectra were referenced with respect to adamantane at 38.48 ppm (relative to neat tetramethylsilane). [45] 11 B MAS NMR experiments were measured using a 16.4-T ( 1 H, 697.8 MHz) Magnex magnet and a home-built spectrometer (David Ruben, FBML-MIT). Experiments were acquired using a 3.2-mm Varian MAS triple-resonance probe, tuned to 11 B. Samples were packed into 3.2 mm (o.d.) ZrO 2 thin-wall rotors (36 μl fill volume). Spectra were acquired using short (20° tip-angle) quantitative pulses, recycle delays of 2 s, between 4096 and 30 720 co-added transients, and a spinning frequency of ω r /2 π =14.00 kHz. All 11 B spectra were referenced using 0.1 M H 3 BO 3 (19.6 ppm) as a secondary standard relative to BF 3 EtO 2 [46] . All XPS spectra were collected using a PHI Versaprobe II equipped with a multichannel hemispherical analyser and aluminium anode X-ray source operating at 100 W with a 100-μm beam scanned over a 1.4-mm line across the sample surface. A dual-beam charge neutralization system was used with an electron neutralizer bias of 1.2 eV and an argon ion beam energy of 10 eV. How to cite this article: Gunther, W.R. et al . Sn-Beta zeolites with borate salts catalyse the epimerization of carbohydrates via an intramolecular carbon shift. Nat. Commun. 3:1109 doi: 10.1038/ncomms2122 (2012).